Crystal structure of an amphiphilic foldamer reveals a 48-mer assembly comprising a hollow truncated octahedron Foldamers provide an attractive medium to test the mechanisms by which biological macromolecules fold into complex three-dimensional structures, and ultimately to design novel protein-like architectures with properties unprecedented in nature. Here, we describe a large cage-like structure formed from an amphiphilic arylamide foldamer crystallized from aqueous solution. Forty-eight copies of the foldamer assemble into a 5-nm cage-like structure, an omnitruncated octahedron filled with well-ordered ice-like water molecules. The assembly is stabilized by a mix of arylamide stacking interaction, hydrogen bonding and hydrophobic forces. The omnitruncated octahedra tessellate to form a cubic crystal. These findings may provide an important step towards the design of nanostructured particles resembling spherical viruses. Nature uses a limited set of amino acids to build proteins that take on a myriad of shapes with defined secondary, tertiary and quaternary structures. In recent years, chemists have shown that this ability to fold into complex structures is not unique to natural biopolymers, and they have begun building ‘foldamers’ comprised of defined sequences of non-natural building blocks that assemble into increasingly complex secondary structures, and even protein-like folds [1] , [2] , [3] . Moreover, foldamers have been designed that are responsive to ligand binding, temperature or that bind to native biologically important proteins, membranes and oligosaccharides [4] , [5] , [6] , [7] , [8] , [9] , [10] , [11] . In this paper, we describe the structural assembly of an amphiphilic arylamide foldamer, 1 ( Fig. 1a ), which assembles into a 48-mer cage-like structure. 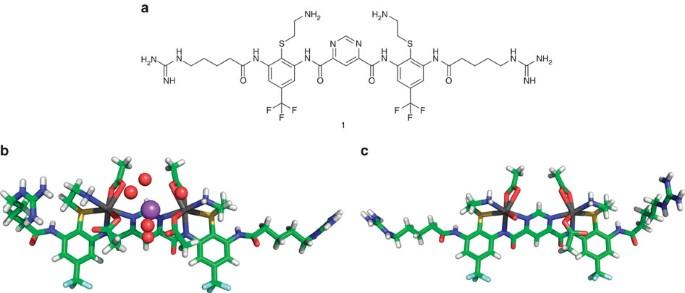Figure 1: Crystal Structure of triarylamide compound 1. (a) The triarylamide compound1. Two monomers in the asymmetric unit have different ligand coordination. (b) Monomer 1 contains two acetates bound to each Cd(II) ion (grey). A hydrated Na+ion (purple sphere) binds between the two Cd(II) sites, maintaining electrical neutrality. (c) Monomer 2 has two acetates bound to one Cd(II), a single acetate bound to the second Cd(II) and no sodium ion. Figure 1: Crystal Structure of triarylamide compound 1. ( a ) The triarylamide compound 1 . Two monomers in the asymmetric unit have different ligand coordination. ( b ) Monomer 1 contains two acetates bound to each Cd(II) ion (grey). A hydrated Na + ion (purple sphere) binds between the two Cd(II) sites, maintaining electrical neutrality. ( c ) Monomer 2 has two acetates bound to one Cd(II), a single acetate bound to the second Cd(II) and no sodium ion. Full size image Compound 1 was originally designed as a mimic of antimicrobial peptides [12] . It is a triarylamide comprising two 1,3-diaminobenzene units linked by a 4,6-dicarboxy-substituted pyrimidine and two terminal guanidine-containing amides. Pendant thioether substituents within the diaminobenzene units help to rigidify the structure and also provide points of attachment for positively charged aminoethyl side chains. Together, these groups create a facially amphiphilic, positively charged structure, previously shown to be essential for their high antibacterial activity in vitro and in animal models [12] . Here we show the crystallographic structure of 1 and confirm its amphiphilic structure, which is required for binding to bilayers. More importantly, the foldamer, which was crystallized from aqueous solution in the absence of membranes, associates to form a honeycomb geometry with each cubicle as a truncated octahedron. The assembly can be understood in terms of physicochemical principles, including the hydrophobic effect, aromatic stacking, hydrogen bonding, and ion-binding and could advance the nanoscale engineering of complex molecular assemblies. Crystal structure of 1 shows the designed amphiphilicity Nuclear magnetic resonance (NMR) studies showed that the triarylamide assembled into a higher order oligomer in aqueous solution ( Supplementary Figs 1 and 2 ). To obtain a high-resolution structure of 1 , it was crystallized from aqueous solution by the hanging-drop method in the presence of 0.05 M cadmium sulphate and sodium acetate (1.0 M). Two monomers with closely related structures form the asymmetric unit ( Fig. 1b,c ). Each monomer shows the expected amphiphilic structure, but the arylamide backbone is stabilized differently in the presence than in the absence of Cd 2+ (ref. 13 ). In the crystal, Cd 2+ ions displace the arylamide protons on the amide units connecting the phenyl and pyrimidyl rings. The foldamers also interact weakly with Cd 2+ in aqueous solution ( Supplementary Fig. 3 ). Each Cd 2+ interacts with the pyrimidyl nitrogen and thioether, replacing the hydrogen-bonded interactions used in the original design with metal–ligand interactions. The neighbouring aminoethyl group serves as a fourth ligand, and acetates or (in one case) a water molecule complete the ligand environment. However there are no ligand–metal ion interactions between sites within a single molecule or between molecules in the crystal lattice. Thus, the metal ions appear to promote crystallization, not by bridging between sites as in assembly systems formed between polycoordinate metal ions and polydentate ligands [14] , but rather by subtly changing the physical and geometric properties of the molecule. The structure of the triarylamide monomer in the crystallographic lattice displays the amphiphilic structure anticipated in the design. The trifluoromethyl groups and the nonpolar portions of the aryl backbone segregate from the strongly polar amine and guanidine side chains. The overall arrangement is consistent with that determined by solid-state NMR of the triarylamide bound to phospholipid bilayers in the absence of Cd 2+ (ref. 15 ). It is unlikely that the metal ion plays a significant role in the biological activity of the molecule, because other variants of this triarylamide that lack the thioether and/or the ethylamine-ligating groups have high antimicrobial activity [7] , [11] . A complex assembly stabilized by diverse interactions The arylamide crystallizes in a space group of high symmetry, P 3 n , which has not yet been seen for an organic framework structure. The unit cell ( Figs 2 and 3 ) contains 24 copies of the asymmetric dimer, arranged in the shape of an omnitruncated octahedron, a special case of an Archimedean solid, the truncated octahedron, which has eight hexagonal and six square faces. Each arylamide dimer associates with 113 water molecules, which are primarily located within the cores of the truncated octahedra, for a total of 2,712 water molecules per unit cell. 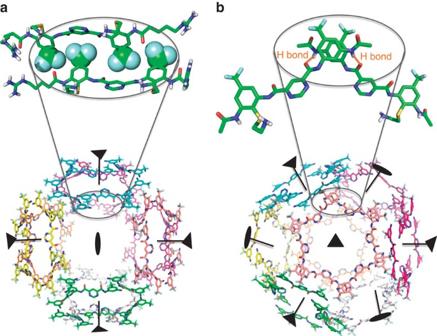Figure 2: Omnitruncated octahedron formed by 48 copies of the triarylamide. (a) The structure is viewed down the square faces, which have twofold symmetry. The hexagonal faces have crystallographic threefold symmetry as shown. The inset shows the packing between arylamide neighbours interacting at edges between hexagonal faces. (b) The structure is viewed down the hexagonal face, which has threefold crystallographic symmetry. The inset shows that the individual arylamides interact with their aryl groups stacked in an offset manner, the adjacent terminal amides in a tight hydrogen bond and the trifluoromethyl groups in close proximity. Figure 2: Omnitruncated octahedron formed by 48 copies of the triarylamide. ( a ) The structure is viewed down the square faces, which have twofold symmetry. The hexagonal faces have crystallographic threefold symmetry as shown. The inset shows the packing between arylamide neighbours interacting at edges between hexagonal faces. ( b ) The structure is viewed down the hexagonal face, which has threefold crystallographic symmetry. The inset shows that the individual arylamides interact with their aryl groups stacked in an offset manner, the adjacent terminal amides in a tight hydrogen bond and the trifluoromethyl groups in close proximity. 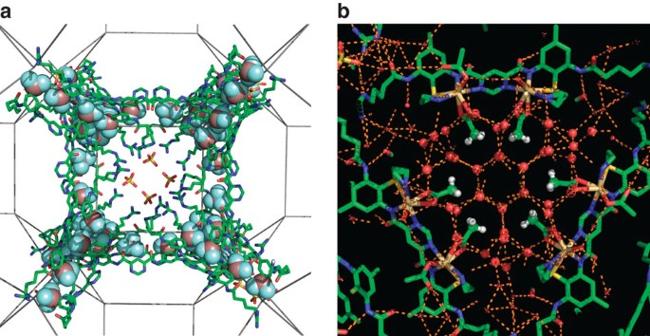Figure 3: Interactions of small molecules and water with the triarylamide. (a) Along the square face, sulphate ions are shown interacting with the Arg-like side chain of the arylamides. Trifluorometyl groups are also shown in space-filling representation; (b) along the square face, the acetates are shown with their methyl groups (protons included) surrounded by a clathrate of water molecules. Full size image Figure 3: Interactions of small molecules and water with the triarylamide. ( a ) Along the square face, sulphate ions are shown interacting with the Arg-like side chain of the arylamides. Trifluorometyl groups are also shown in space-filling representation; ( b ) along the square face, the acetates are shown with their methyl groups (protons included) surrounded by a clathrate of water molecules. Full size image The 48 triarylamides lie with their backbones roughly parallel to the edges of the eight hexagons ( Fig. 2 ). Each arylamide engages in two distinct types of interactions, which together uniquely define and stabilize the overall assembly. Arylamides that lie along the edges of neighbouring hexagons interact in what we term a ‘trifluoromethyl zipper’ interaction, in which the water-repelling trifluoromethyl groups intimately interdigitate along a non-exact twofold axis of symmetry. This trifluoromethyl zipper arrangement is reminiscent of the leucine zippers [16] that stabilize coiled coils in water-soluble proteins, as well as the alanine coils found frequently in membrane proteins [17] . While engaging in trifluoromethyl zipper interactions, the arylamides also engage in a second type of interaction between arylamides that lie within a single hexameric ring. We designate this interaction as the arylamide elbow motif; the terminal phenyl rings of the arylamides in this motif stack in a face-to-face interaction with the centers of the rings offset as often seen in aromatic stacking [18] . The dimer is further stabilized by tight hydrogen bonding between the terminal amide groups, and their trifluoromethyl groups also cluster together. The hydrogen-bonded interaction between meta-substituted amides leads to a 120° angle between the two arylamides, which is repeated to create the hexameric rings. The simultaneous interactions of the triarylamides in both the trifuoromethyl zipper and the arylamide elbow motif create the 48-mer assembly seen in the crystal ( Fig. 2 ). The arylamide elbows create the hexamers, while the trifluoromethyl zippers couple adjacent hexamers to form the overall three-dimensional structure. Interestingly, this arrangement also leads to extensive clustering of the trifluoromethyl groups along the vertices, creating fluorocarbon cores ( Fig. 3a ). Electrostatic and hydrogen-bonded interactions between sulphate ions and the arginine-like guanidine side chains feature prominently in each four-sided face of the truncated octahedron ( Fig. 3 ). A total of four sulphates are seen in each face, two coming from each unit cell of the crystal lattice ( Fig. 3a ). Each sulphate receives a total of six hydrogen bonds from three guanidine-containing side chains that engage the anion in a bidentate interaction. The hexagonal faces also show a rich array of molecular interactions; the methyl groups of the acetates (counterions of the Cd 2+ ions) project towards the center of the hexagon ( Fig. 3b ). Each acetate ion is surrounded by a clathrate of water molecules, which join near the center to create a nearly ideal ice-like hexagon of water molecules. The individual truncated octahedra found in the unit cell tessellate in three dimensions to form a cube. Intersecting square and hexagonal channels run through the length of the crystal ( Fig. 4 ). Arylamides that do not form a trifluoromethyl zipper within an individual unit cell, form an equivalent zipper motif with other monomers from adjacent unit cells. Also, the packing of the truncated octahedra contribute to the cluster of sulphate/guanidine interactions along the square channels, as well as the clustering of trifluoromethyl groups at the vertices and along the hexagonal channels. Thus, the same interactions that stabilize individual truncated octahedra also contribute to their packing into a crystal lattice. 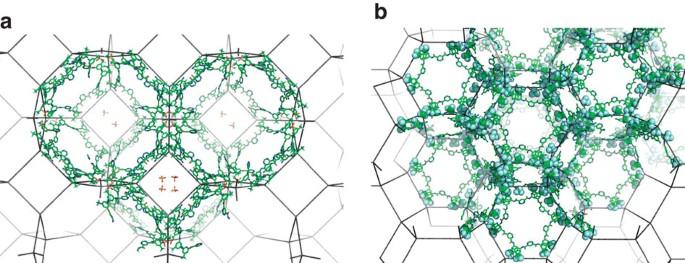Figure 4: Packing of the unit cells in the crystal structure. Three-dimensional space is compactly packed by the unit cells, viewed down the square (a) and hexagonal (b) channels. Figure 4: Packing of the unit cells in the crystal structure. Three-dimensional space is compactly packed by the unit cells, viewed down the square ( a ) and hexagonal ( b ) channels. Full size image Assembly of compound 1 in aqueous solution To determine how the compound behaves in solution, we also performed NMR and ultraviolet–visible spectroscopy experiments in a buffer similar to the crystallization solution. Proton assignments for the peaks resonating between 7.0 and 10.0 p.p.m. are obtained by one-dimensional and two-dimensional NMR ( Supplementary Fig. 1 ). NMR titration of the compound with Cd 2+ ions ( Supplementary Fig. 2 ) shows that on addition of metal ion the peaks were broadened and in some cases appear at new positions in the spectrum. At substoichiometric Cd 2+ concentrations, multiple peaks are observed, indicating that different forms of 1 with 0, 1 and 2 equivalents of Cd 2+ bound were in slow-to-intermediate exchange on the time scale of the differences in chemical shift between the various forms (micro to milliseconds). After a stoichiometric amount (two equivalents per foldamer) of Cd 2+ is reached, the peaks begin sharpening as the distribution becomes more homogeneous. Little change is observed after 5.0 equivalents (40 mM) were added. These data show that the foldamer binds Cd 2+ stoichiometrically at this concentration, and that it existed in the Cd 2+ -bound state under conditions of crystallization. Also, ultraviolet–visible spectroscopy confirmed that Cd 2+ binds to the foldamer in a 2:1 (metal ion/foldamer) stoichiometry, as in the crystal ( Supplementary Fig. 3 ). To examine the self-association of the foldamer, we examined the concentration dependence of its proton and 19 F NMR spectra while holding the Cd 2+ constant at saturating concentrations. As the concentration was increased to 2 mM the proton NMR spectra showed small changes, while at 8.2 mM the peaks shifted further and two new peaks appeared in the spectrum ( Fig. 5a ). The new peaks are assigned to amides and guanidine protons from 1 , as was confirmed by hydrogen-deuterium exchange ( Fig. 5b ). The fact that, at the highest concentration, the amides were observable at pH 7.5 in H 2 O shows that their exchange with bulk solvent is slowed by the formation of an oligomer. The concentration-dependent 19 F NMR spectra also showed biphasic changes ( Fig. 5c ). In this case, larger changes in chemical shift were observed between 0.1 and 2 mM. A second process occurs at higher concentrations (between 2 and 10 mM), causing the peaks to shift in the reverse direction and to broaden. While a quantitative analysis is complicated by the many equilibria, these data clearly show that 1 associates in aqueous solution, and that the mean association state increases as the concentration increases. 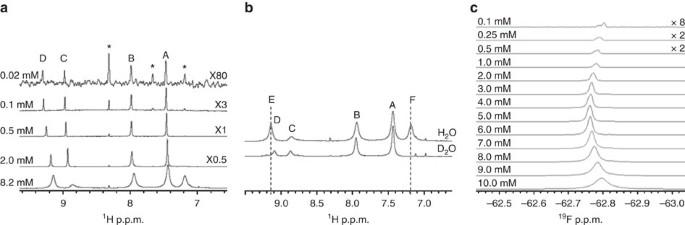Figure 5: NMR studies on the foldamer 1. (a)1H NMR spectra as a function of the concentration of1(298 K, 95% H2O/5% D2O, 30 mM CdSO4, 100 mM HEPES pH 7.5 and 600 mM NaOAc). (b) Comparison of the same sample recorded in H2O and D2O shows the disappeared exchangeable protons E and F in D2O highlighted by the dash lines. The H2O sample was 8.2 mM compound in 30 mM cadmium sulphate, 100 mM HEPES pH 7.5, 600 mM sodium acetate and the D2O sample was obtained by lyophilizing the H2O sample overnight and then adding D2O. (c)19F NMR spectra as a function of concentration of1at 95% H2O/5% D2O, 100 mM HEPES pH 7.5, 1 M NaOAc and 50 mM CdSO4. Assignments for protons A–F are given inSupplementary Figs 1 and 2. Peaks labelled with a * are impurities in the buffer. Figure 5: NMR studies on the foldamer 1. ( a ) 1 H NMR spectra as a function of the concentration of 1 (298 K, 95% H 2 O/5% D 2 O, 30 mM CdSO 4 , 100 mM HEPES pH 7.5 and 600 mM NaOAc). ( b ) Comparison of the same sample recorded in H 2 O and D 2 O shows the disappeared exchangeable protons E and F in D 2 O highlighted by the dash lines. The H 2 O sample was 8.2 mM compound in 30 mM cadmium sulphate, 100 mM HEPES pH 7.5, 600 mM sodium acetate and the D 2 O sample was obtained by lyophilizing the H 2 O sample overnight and then adding D 2 O. ( c ) 19 F NMR spectra as a function of concentration of 1 at 95% H 2 O/5% D 2 O, 100 mM HEPES pH 7.5, 1 M NaOAc and 50 mM CdSO 4 . Assignments for protons A–F are given in Supplementary Figs 1 and 2 . Peaks labelled with a * are impurities in the buffer. Full size image Proteins are built up from secondary structures with a pronounced facially amphiphilic character, which have also served as building blocks in the design of the first helical bundles composed of peptides synthesized from both α- and β-amino acids. Therefore, it was of considerable interest to determine the structures formed by the present triarylamides. The discovery of a large cage-like structure is interesting, given the complex protein-like interactions that stabilize the assembly. It is of interest to compare the observed structure of 1 with those more purposefully designed, built from proteins [19] , [20] , [21] or small molecules [14] . Organic crystals are often assembled through strong directional intermolecular forces in organic solvents [22] . One of the most active fields in crystal engineering is metal-organic frameworks, assembly systems with predetermined directionalities between polycoordinate metal ions and polydentate ligands [14] . In addition, certain organic frameworks are built by strong hydrogen bonding [23] . The assembly described here uses a diversity of interactions similar to those employed by natural proteins. It is also interesting to consider its construction in terms of ‘supramolecular synthons’, as in other examples of crystal engineering. The arylamide elbow motif in triarylamide can be considered a supramolecular synthon, which engages in both hydrogen bonding and aromatic stacking ( Fig. 6a , in pink shadow). The two N-H···O=C hydrogen bonds in the arylamide elbow motif have a distance of 2.8 Å and an angle of 157° and 166°, which show that they are strong hydrogen bonds as in other examples of crystal engineering [24] . The distance between the two phenyl rings is 3.7 Å, as observed in other crystal studies [25] . Moreover, the pronounced facially amphiphilic character and high symmetry of 1 gives rise to its assembly and crystallization into an omnitruncated octahedron in aqueous environments. The assembly can be conceptually analysed according to Aufbau principles [26] , although the complexity of its structure and self-association equilibria before crystallization render it difficult to assign a detailed kinetic mechanism of assembly. Hydrogen bonding and aromatic stacking provide geometrically specific interactions that stabilize the aromatic elbow ( Fig. 6a ), and repetition of this interaction pattern leads to assembly of the hexameric ring ( Fig. 6b ) that forms the hexagonal face of the truncated octahedron. Two hexagons can further assemble via hydrophobic association of trifluoromethyl groups, and hydrogen bonding between the guanidine and carbonyl of neighbouring arginine-like groups stabilize ( Fig. 6c ). The formation of the solvent-inaccesible trifluoromethyl core is further consolidated by the assembly of two more hexagons; the resulting saddle-shaped tetramer of hexamers forms a complete vertex for the truncated octahedron ( Fig. 6d ). Two such tetramers of hexamers associate and create a double crown assembly on the square face ( Fig. 6e ), which serves as a long-range synthon module, for packing in the late stages of crystallization [27] . This supramolecular subunit packs in primitive cubic cells and generates a crystalline framework ( Fig. 6f ). 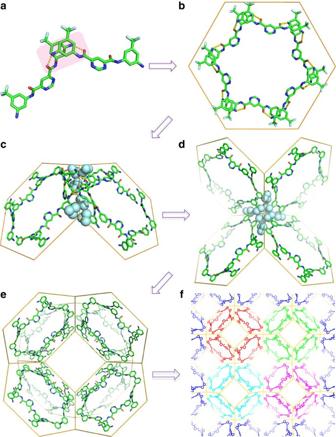Figure 6: Hierarchical assembly of the foldamer crystal. Hydrogen bonds are shown as yellow dashed lines and fluorine atoms are displayed as spheres. The yellow wires are lattices defined by the symmetry of the crystal. (a) The supramolecular synthon (denoted in pink shadow) is characterized by its combined aromatic and hydrogen-bonding interactions. (b) The elbow-like synthons induce the formation of a hexagonal ring. (c) Two six-membered rings associate by hydrophobic trifluoromethyl zippers and hydrogen bonds between the guanidine and carbonyl. (d,e) Further stabilization by trifluoromethyl zippers prompts the assembly of a saddle-shaped tetramer of hexamers and then the double-crown-shaped long-range synthon module. (f) The modules pack in primitive cubic cells to form the framework-like crystal. Figure 6: Hierarchical assembly of the foldamer crystal. Hydrogen bonds are shown as yellow dashed lines and fluorine atoms are displayed as spheres. The yellow wires are lattices defined by the symmetry of the crystal. ( a ) The supramolecular synthon (denoted in pink shadow) is characterized by its combined aromatic and hydrogen-bonding interactions. ( b ) The elbow-like synthons induce the formation of a hexagonal ring. ( c ) Two six-membered rings associate by hydrophobic trifluoromethyl zippers and hydrogen bonds between the guanidine and carbonyl. ( d , e ) Further stabilization by trifluoromethyl zippers prompts the assembly of a saddle-shaped tetramer of hexamers and then the double-crown-shaped long-range synthon module. ( f ) The modules pack in primitive cubic cells to form the framework-like crystal. Full size image In conclusion, the crystallographic structure of 1 has revealed a visually arresting Archimedean solid. The interactions that stabilize this assembly are readily apparent and should encourage future rational designs of foldamers with well-defined tertiary and quaternary structures. Crystallography The arylamide foldamer 1 was synthesized, as described previously [12] , and dissolved at 20 mg ml −1 in water. Crystals were obtained using the hanging-drop vapor-diffusion method at room temperature, by mixing equal volumes of foldamer solution with reservoir solution containing 0.05 M CdSO4, 0.1 M HEPES pH 7.5 and 1.0 M NaOAc. Crystals were flash frozen with the cryoprotectant Parabar 10312 (Hampton Research), and data to 0.920 Å were collected on the beamlines 24-ID-E and 24-ID-C at Advanced Photon Source, Argonne National Laboratory. The structure was solved by direct methods, as described in the Supplementary Methods . NMR spectroscopy Spectra were recorded at 298 K on a Bruker 800 or 900 MHz spectrometer equipped with a cryogenic probe for 1 H spectra or a Bruker 300 MHz for 19 F spectra. 1 H spectra typically were recorded with 256 scans and 31 p.p.m. spectral width and 19 F spectra typically were recorded with 256 scans and 100 p.p.m. spectral width. 1 H chemical shifts were referenced with respect to the residual water peak at 4.75 p.p.m. and the 19 F chemical shifts were calibrated using the external standard trifluoroacetic acid chemical shifts at −76.6 p.p.m. All spectra were processed and analysed using the program TopSpin 3.0 (Bruker, Karlsruhe, Germany). Before Fourier transformation, time domain data were multiplied by sine square bell window functions shifted by 90° and zero-filled once. Additional details are provided in Supplementary Methods . How to cite this article: Pavone, V. et al . Crystal structure of an amphiphilic foldamer reveals a 48-mer assembly comprising a hollow truncated octahedron. Nat. Commun. 5:3581 doi: 10.1038/ncomms4581 (2014). Accession codes : Crystal structure for the triarylamide can be accessed from the Cambridge Crystallographic Data Centre (CCDC) with Deposition number 956538. These data can be obtained free of charge from The Cambridge Crystallographic Data Centre via www.ccdc.cam.ac.uk/data_request/cif .